Complete architecture of the archaeal RNA polymerase open complex from single-molecule FRET and NPS The molecular architecture of RNAP II-like transcription initiation complexes remains opaque due to its conformational flexibility and size. Here we report the three-dimensional architecture of the complete open complex (OC) composed of the promoter DNA, TATA box-binding protein (TBP), transcription factor B (TFB), transcription factor E (TFE) and the 12-subunit RNA polymerase (RNAP) from Methanocaldococcus jannaschii . By combining single-molecule Förster resonance energy transfer and the Bayesian parameter estimation-based Nano-Positioning System analysis, we model the entire archaeal OC, which elucidates the path of the non-template DNA (ntDNA) strand and interaction sites of the transcription factors with the RNAP. Compared with models of the eukaryotic OC, the TATA DNA region with TBP and TFB is positioned closer to the surface of the RNAP, likely providing the mechanism by which DNA melting can occur in a minimal factor configuration, without the dedicated translocase/helicase encoding factor TFIIH. Transcription of all cellular genomes is carried out by evolutionary related multisubunit RNA polymerases (RNAPs). In contrast to eukaryotes, where different types of RNAPs exist, archaea utilize only one RNAP to transcribe their genes, but its subunit composition, structure and utilization of general transcription factors is strikingly similar to the eukaryotic RNAP II (Pol II) system [1] , [2] . Eukaryotic Pol II involves the interplay of a large set of transcription factors to initiate transcription, most importantly general transcription factors TFIIA, B, D, E, F and H. However, not all factors are strictly required; in particular TFIIA is only necessary to alleviate the repressive effects of negative regulators such as NC1. Moreover, using strong promoters and negatively supercoiled DNA templates only two factors TATA box-binding protein (TBP) and TFIIB suffice to direct start site specific transcription initiation by Pol II in vitro [3] . TBP and TFIIB assemble at the promoter [4] and recruit Pol II as well as other factors to form the preinitiation complex (PIC). This complex is referred to as the closed complex (CC), which subsequently undergoes large conformational rearrangements during which the DNA strands are separated and the template DNA strand (tDNA) is loaded into the RNAP active site to form the open complex (OC). In eukaryotes, this process is greatly enhanced by the helicase activities encoded by TFIIH. The large size, heterogeneous composition and conformationally dynamic nature of eukaryotic PICs have made their structural and functional analysis problematic. Recent advances in the field have improved our understanding of the overall structural organization of the eukaryotic PIC. X-ray structures of PIC sub-complexes (encompassing Pol II and TFIIB fragments) at high resolution have provided hints of mechanistic aspects of the CC-to-OC transition during transcription initiation. Thus the crystal structure of the Pol II–TFIIB complex allowed for modelling of the CC and OC [5] , [6] , [7] . Several crosslinking studies have yielded information about the location of transcription factors TFIIB [8] , TFIIF, TFIIE [9] , [10] and TFIIH [11] . Recent cryo-electron microscopy (cryo-EM) studies have provided overall structures of both the eukaryotic and archaeal PICs at low to intermediate resolution [12] , [13] , [14] . However, all of these studies have failed to fully resolve the course of the DNA within the OC, likely due to the flexibility of the transcription bubble. The archaeal transcription apparatus is an excellent model system for the eukaryotic Pol II system [15] as its RNAP and associated basal transcription factors are homologous, and because the entire system from hyperthermophilic archaea can be reconstituted from recombinant proteins [16] . This enables us to site specifically introduce mutations or molecular probes such as fluorescent dyes for single-molecule fluorescence analysis [17] , [18] . The factors TBP and transcription factor B (TFB; homologous to TFIIB) are necessary and sufficient for promoter-directed start site-specific transcription initiation of the archaeal RNAP, which mirrors the minimal factor requirements for Pol II (refs 3 , 16 , 19 ). A third factor, TFE (homologous to TFIIEα) interacts with RNAP and stimulates OC formation, also comparable to the Pol II system [18] , [20] , [21] , [22] . The pivotal difference between the two systems is the apparent ease at which the OC is formed in archaea, whereas in eukaryotes the additional helicase/translocase activity of the general factor TFIIH is required in vivo , which is not conserved in any archaeal species. Single-molecule techniques have shown great potential to resolve the dynamics of transcription processes because they allow for the direct and real-time observation of transcription, one molecule at a time [23] . To obtain quantitative structural and dynamic information about transcription complexes during various phases of transcription, the Nano-Positioning System (NPS) was developed [24] . The NPS combines data from single-molecule Förster resonance energy transfer (smFRET) measurements with existing structural information and a rigorous analysis using Bayesian parameter estimation. As a result, three-dimensional probability density functions for dye molecules (‘antennas’) attached to positions in unknown, flexible regions of the complex of interest can be calculated. For visualization, the smallest volume enclosing a certain probability of the computed density, the credible volume, can be displayed together with the known structure. The recorded smFRET data are measured between the antennas and dye molecule (‘satellites’) attached to known positions from the crystal structure [24] . This method has been used in Pol II transcription elongation complexes (ECs) to study the position of the exiting RNA [25] , the influence of transcription factor TFIIB on the position of the nascent RNA [24] and the position of non-template DNA (ntDNA) and upstream DNA [26] . Moreover, the architecture of a minimal Pol II OC [27] and the position of transcription factor TFE in the archaeal PIC [18] have been determined. NPS has been further extended to a global analysis where a complete data set of all measured information about all the antenna-satellite pairs is used as a network to simultaneously infer the position of all the antennas [28] . Here, we used smFRET, global NPS analysis and fluorescently labelled components of the transcription machinery from the hyperthermophilic archaeon Methanocaldococcus jannaschii (Mj) to determine the molecular architecture of the complete archaeal OC consisting of RNAP, promoter DNA, TBP, TFB and TFE. We determined the smFRET efficiencies between unknown ‘antenna’ dye molecules and several known ‘satellite’ dye molecules incorporated at one of five reference sites in the RNAP, whose position can be inferred from crystallographic structures. The ‘antenna’ dyes are attached to either one of several positions on the upstream and downstream ntDNA strand to TBP or to TFB. The probability densities generated from the NPS calculation allow us to build a model of the complete archaeal OC, which provides valuable insights into the mechanism of transcription initiation. We find the two factors TBP and TFB to be located closer to the RNAP surface in archaeal complexes compared with the Pol II system. This can provide an answer to the question why the CC-to-OC transition readily occurs in archaea but necessitates TFIIH in the Pol II system, thus illustrating how during evolution of the eukaryotic domain of life subtle changes in the architecture of the initiation complex renders DNA melting largely dependent on TFIIH. Assembly of well defined OCs for smFRET experiments Complete archaeal OCs were assembled using M. jannaschii TBP (MjTBP), TFB, TFE and RNAP (Methods) on the strong SSV T6 promoter as DNA template. To ensure that the complexes were in the open state, a non-complementary four nucleotide ‘mismatch’ was introduced in the promoter [16] , [29] . To perform smFRET experiments, the complexes were labelled with a fluorescent donor and acceptor at desired locations. Fluorescently labelled DNA oligonucleotides, TBP, TFB, TFE and RNAP were combined to yield a large network of ~70 differently labelled complexes, each with a single smFRET pair at a desired location ( Fig. 1a,b ). Previous biochemical studies had established the formation of stable OCs from these components, capable of promoter-specific transcription initiation in vitro , forming RNA templates from a precise starting point (+1; ref. 22 ). Complex formation of this in vitro OC was also verified by electrophoretic mobility shift assays [18] . 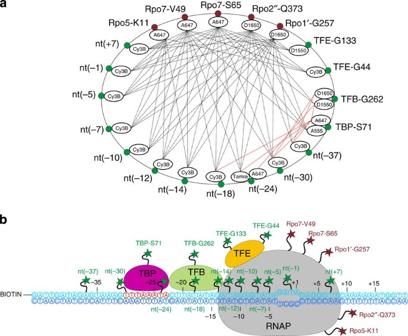Figure 1: Schematic representation of the global FRET network. (a) All unknown antenna positions (green circles) and the five known satellite sites on the RNAP (dark red circles) are shown together with the corresponding attached dyes (A647=Alexa 647; A555=Alexa555; Dl550=DyLight550; Dl650=DyLight650). FRET efficiencies were measured between pairs of satellite (acceptor) and antenna (donor) dyes (dotted black lines) and in between antennas (dotted red lines). In case of the latter measurements, one of the antenna positions had to be labelled with an acceptor, as indicated. (b) Cartoon depicting the mismatched (−3 to +1) viral SSV T6 promoter (tDNA in blue, ntDNA in cyan, TATA box in red), which is used throughout this study51. Labelling sites on the DNA and on the transcription factors TBP, TFB and TFE are marked with a green star. Labelling sites on the RNAP are marked with a dark red star. Proteins contained within the archaeal OC are shown schematically. See alsoSupplementary Figs 1,2 and 4. Figure 1: Schematic representation of the global FRET network. ( a ) All unknown antenna positions (green circles) and the five known satellite sites on the RNAP (dark red circles) are shown together with the corresponding attached dyes (A647=Alexa 647; A555=Alexa555; Dl550=DyLight550; Dl650=DyLight650). FRET efficiencies were measured between pairs of satellite (acceptor) and antenna (donor) dyes (dotted black lines) and in between antennas (dotted red lines). In case of the latter measurements, one of the antenna positions had to be labelled with an acceptor, as indicated. ( b ) Cartoon depicting the mismatched (−3 to +1) viral SSV T6 promoter (tDNA in blue, ntDNA in cyan, TATA box in red), which is used throughout this study [51] . Labelling sites on the DNA and on the transcription factors TBP, TFB and TFE are marked with a green star. Labelling sites on the RNAP are marked with a dark red star. Proteins contained within the archaeal OC are shown schematically. See also Supplementary Figs 1,2 and 4 . Full size image While smFRET experiments can reveal both the structure and dynamics of macromolecular complexes, they only focus on one smFRET value of one dye pair at a time. Therefore, it is important to ensure that complexes are formed properly and that the information obtained from the measurement is indicative of the desired complex. To this end, we performed a number of control experiments ( Supplementary Methods ). We found that stable OCs were formed in a factor-dependent manner ( Supplementary Fig. 1a,b ) but that transcription factor TFE did not exert an influence on the architecture of the OC ( Supplementary Fig. 2a–d ). Also, we found that the choice of the dye on the DNA strand had no effect on the distance information obtained from smFRET experiments ( Supplementary Fig. 2e ). OCs with the tDNA strand at the active centre In contrast to the ntDNA strand, the position of the tDNA strand of the melted region in the OC could be inferred from the crystal structure of yeast Pol II using a tailed DNA template [30] . The position of the tDNA strand resembles that of the respective EC, even in the absence of RNA [31] . To build the model of the eukaryotic OC, DNA opening was assumed to commence 20 bp downstream of TATA [32] , yielding a DNA melted in a region between positions (+2) to (−13) (ref. 5 ). To ascertain that the extent of the melted region in the M. jannaschii OC was comparable to the published data of the Pyrococcus system [33] , [34] , we used KMnO 4 footprinting ( Supplementary Fig. 3 and Methods). This method detects thymidine nucleobases in single-stranded DNA regions. The SSV T6 promoter template contains a mismatch region from (−3) to (+1) and thus contains an obligate single-stranded T at register (−1). This residue serves as a positive control and is detectable in the free promoter probe. Addition of TBP, TFB and RNAP leads to novel signals at register (−5) and (−7), reflecting the opening of the promoter by the transcription complex. Since the next T residue occurs at (−12), we conclude that the transcription bubble starts at (−1) extends to at least (−7) and importantly not beyond (−12), showing that the size of the melted region in our OC is in good agreement with the published results for the Pyrococcus system [33] . Since pre-opened promoter templates were used, the transcription factor TFE did not significantly alter DNA melting and did not exert an influence on the architecture of the OC ( Supplementary Figs 2 and 3 ). Furthermore, we tested whether the tDNA strand was properly loaded into the active centre cleft. Therefore, we used NPS to localize two dye positions on the tDNA strand, namely tDNA(+3) and tDNA(−9) (Methods, Fig. 2a ). For each position, we performed a set of smFRET measurements with a second dye molecule attached to one of the five reference sites on the RNAP: residue 257 of Rpo1′, residue 373 of Rpo2″, residue 11 of Rpo5, residues 49 and 65 of Rpo7 ( Fig. 2a , Supplementary Fig. 4 and Methods). Exemplary histograms are shown for position tDNA(−9) ( Fig. 2b–f ) and the extracted data are summarized in Supplementary Table 1 . 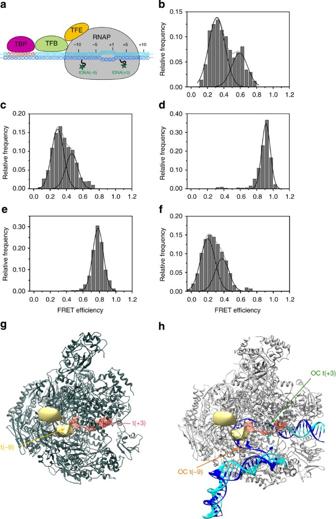Figure 2: Localization of two positions on the tDNA strand in the archaeal OC. (a) Cartoon depicting the labelling positions on the tDNA strand, which were localized using the NPS (colour coding according toFig. 1). (b–f) Frame-wise smFRET histograms used in the NPS localization of tDNA(−9). Shown is the smFRET data from measurements between tDNA(−9) and Rpo7-V49 (b), Rpo7-S65 (c), Rpo2″-Q373 (d), Rpo1′-G257 (e) and Rpo5-K11 (f), respectively. The histograms were fitted with a double (b,c,f) or single (d,e) Gaussian distribution indicated by the black lines. In (b,c,f) the grey line represents the sum of the two Gaussian distributions. Results of the fits together with those obtained during localization of tDNA(+3) are summarized in Supplementary Table 1. (g) NPS results for the fluorescent probes attached to tDNA(+3) (pink) and tDNA(−9) (yellow). The X-ray structure of the archaeal polymerase ofS. shibatae(PDB: 2WAQ)37is represented as dark grey ribbon. Note, that at this confidence level, the credible volume of tDNA(−9) is divided into two areas, if the credible volume is drawn at higher confidence these two areas merge (see text for details). (h) Comparison of the NPS results to the eukaryotic open complex model5. The X-ray structure of the yeast polymerase is represented as light grey ribbon, the tDNA is shown in blue and the ntDNA is shown in cyan. The corresponding eukaryotic bases for tDNA(+3) (green) and tDNA(−9) (orange) are encircled. The NPS credible volumes are in good agreement to the model. See alsoSupplementary Fig. 3. Figure 2: Localization of two positions on the tDNA strand in the archaeal OC. ( a ) Cartoon depicting the labelling positions on the tDNA strand, which were localized using the NPS (colour coding according to Fig. 1 ). ( b – f ) Frame-wise smFRET histograms used in the NPS localization of tDNA(−9). Shown is the smFRET data from measurements between tDNA(−9) and Rpo7-V49 ( b ), Rpo7-S65 ( c ), Rpo2″-Q373 ( d ), Rpo1′-G257 ( e ) and Rpo5-K11 ( f ), respectively. The histograms were fitted with a double ( b , c , f ) or single ( d , e ) Gaussian distribution indicated by the black lines. In ( b , c , f ) the grey line represents the sum of the two Gaussian distributions. Results of the fits together with those obtained during localization of tDNA(+3) are summarized in Supplementary Table 1. ( g ) NPS results for the fluorescent probes attached to tDNA(+3) (pink) and tDNA(−9) (yellow). The X-ray structure of the archaeal polymerase of S. shibatae (PDB: 2WAQ) [37] is represented as dark grey ribbon. Note, that at this confidence level, the credible volume of tDNA(−9) is divided into two areas, if the credible volume is drawn at higher confidence these two areas merge (see text for details). ( h ) Comparison of the NPS results to the eukaryotic open complex model [5] . The X-ray structure of the yeast polymerase is represented as light grey ribbon, the tDNA is shown in blue and the ntDNA is shown in cyan. The corresponding eukaryotic bases for tDNA(+3) (green) and tDNA(−9) (orange) are encircled. The NPS credible volumes are in good agreement to the model. See also Supplementary Fig. 3 . Full size image Many of the observed smFRET histograms showed a secondary peak with a relative intensity varying between 5–30%. However, there was no evidence for dynamic interconversion between the two peaks. Instead, the side peak is likely caused by a different static population. Comparison of NPS analysis of side peaks and main peaks showed only minor changes in credible volume position ( Supplementary Fig. 5 ). In the following, we restrict ourselves to the discussion of the main peaks; however, one should note that, while the side peaks would lead to small Angstrom level alterations of the model, the general conclusions of this work are not affected. The use of Bayesian parameter estimation allows the computation of the most likely position and the three-dimensional uncertainty of the position of the fluorescent dye attached to the unknown position [24] . For this, the uncertainties due to the presence of flexible linkers between the dye and the known positions on the RNAP were computed first ( Supplementary Fig. 4 and Methods). Moreover, for each dye pair, we experimentally determined the fluorescence anisotropies and the isotropic Förster radii (Methods and Supplementary Table 2 ). 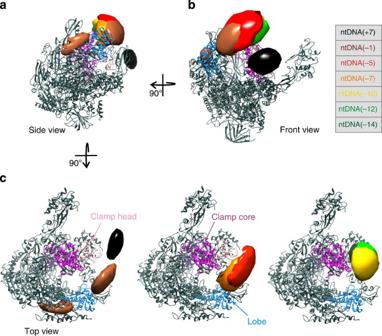Figure 3: Localization of the ntDNA strand in the archaeal OC. (a,b) Side and front view of the archaeal RNA polymerase including the NPS results for the fluorescent probes attached to ntDNA(+7) (black), ntDNA(−1) (brown), ntDNA(−5) (red), ntDNA(−7) (orange), ntDNA(−10) (yellow), ntDNA(−12) (green) and ntDNA(−14) (dark green, hardly visible). (c) Top view (slightly rotated for a clearer view) of archaeal RNA polymerase with selective volumes shown at a time for clarity. See alsoSupplementary Figs 2 and 6. Three-dimensional probability densities were then calculated using the respective linker lengths and the sizes of the dye molecules ( Supplementary Table 3 ) and credible volumes were calculated and displayed in comparison with the crystal structure of the RNAP ( Fig. 2g,h ). The size of all credible volumes presented in this study corresponds to 68% credibility, representing the smallest volume, which encloses a probability of 68%. The credible volume of the dye attached to tDNA(+3) is located inside the cleft, in good agreement with the eukaryotic OC models [5] , [27] . Also tDNA(−9) localizes at a position consistent to the eukaryotic OC models and the position is distinct from the one it would adopt in a CC conformation [5] ( Fig. 2h ). In the case of tDNA(−9), the displayed volume is split into two distinct sub-volumes. One should note that this is not originating from the dynamic movement between these positions (our model is a static model) but represents the positioning uncertainty of this DNA position in the calculation at 68% confidence level. In fact, if drawn at higher confidence the two volumes merge. The path of the ntDNA strand within the archaeal OC To determine the path of the ntDNA strand, we assembled a variety of OCs, where a fluorescent donor dye was attached to ntDNA(+7), (−1), (−5), (−7), (−10), (−12) or (−14) (Methods). For each of these ntDNA fluorescent donor positions, a fluorescent acceptor was attached to one of the five different reference sites on the RNAP, generating five unique complexes per labelled donor position. Exemplary histograms are shown ( Supplementary Fig. 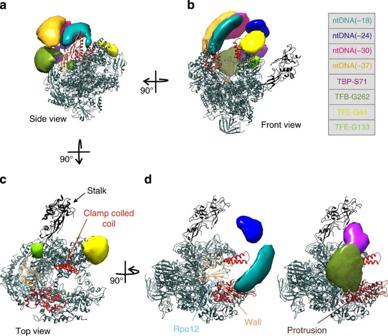Figure 4: Localization of the TATA DNA and transcription factors in the archaeal OC. (a,b) Side and front view of the archaeal RNA polymerase together with the NPS results for the fluorescent probes attached to ntDNA(−18) (dark cyan), ntDNA(−24) (dark blue), ntDNA(−30) (magenta), ntDNA(−37) (gold), TBP-S71 (purple), TFB-G262 (olive), TFE-G44 (yellow) and TFE-G133 (green). (c) Top view of archaeal RNA polymerase with only the NPS credible volumes TFE-G44 (yellow) and TFE-G133 (green) shown at a time to illustrate their proximity to the clamp coiled-coil region of subunit Rpo1′ (red) and to the stalk of the RNAP (black), respectively. (d) Alternative view obtained by a 90° rotation of the top view, showing the proximity of the NPS credible volume ntDNA(−18) (dark cyan) to the protrusion (brown) of subunit Rpo2″. The NPS credible volume of ntDNA(−24) (dark blue) is situated further away from the RNAP surface compared with the position of ntDNA(−18). Also, the proximity of the NPS credible volumes TBP-S71 (purple) and TFB-G262 (olive) to the wall domain (beige) of subunit Rpo2″ and to subunit Rpo12 (light blue) can be seen. The volume of TFB-G262 is made transparent for clarity. See alsoSupplementary Figs 6 and 7. 6b–f ) and the extracted data are summarized in Supplementary Table 4 . In the global NPS analysis [28] , the complete data set consisting of mean FRET efficiencies, dye attachment information (position, length of linker and size of dye molecule), steady state fluorescence anisotropies and isotropic Förster distances of all antenna-satellite pairs and the uncertainty in position of the satellite dyes (due to linker length and dye molecule size) were used to simultaneously infer the positions of all antennas within the RNAP coordinate system ( Fig. 1 and Methods). As a result of Bayesian parameter estimation, we obtained the three-dimensional probability density of each antenna, which represents the position of the dye attached to the DNA base ( Fig. 3a–c ). Figure 3: Localization of the ntDNA strand in the archaeal OC. ( a , b ) Side and front view of the archaeal RNA polymerase including the NPS results for the fluorescent probes attached to ntDNA(+7) (black), ntDNA(−1) (brown), ntDNA(−5) (red), ntDNA(−7) (orange), ntDNA(−10) (yellow), ntDNA(−12) (green) and ntDNA(−14) (dark green, hardly visible). ( c ) Top view (slightly rotated for a clearer view) of archaeal RNA polymerase with selective volumes shown at a time for clarity. See also Supplementary Figs 2 and 6 . Full size image The furthest downstream position was ntDNA(+7) in the downstream duplex region. The NPS credible volume is located close to the clamp head region of subunit Rpo1′ but outside of the cleft ( Fig. 3c , black). NtDNA(−1) lies within the single-stranded region of the ntDNA strand and its position ( Fig. 3c , brown) is split into two distinct sub-volumes located at the edge of the cleft, proximal to the lobe domain of subunit Rpo2″. As for tDNA(−9), these sub-volumes are not originating from dynamic movement but represent the uncertainty in position at 68% confidence level; if drawn at higher confidence the two volumes would merge. The positions of the dye molecules attached to the next upstream bases ntDNA(−5) ( Fig. 3c , red) and ntDNA(−7) ( Fig. 3c , orange) occupy a similar region within the cleft, between the clamp core of subunit Rpo1′ and the lobe domain of Rpo2″. The position of ntDNA(−10) ( Fig. 3c , yellow) is located closer to the clamp coiled-coil region of subunit Rpo1′. The volumes for ntDNA(−12) ( Fig. 3c , green) and ntDNA (−14) ( Fig. 3c , dark green, hardly visible) are largely overlapping and remain at the same side of the clamp coiled-coil region as ntDNA(−10). We repeated the NPS calculation with a slightly modified crystal structure of the archaeal RNAP, where we moved the clamp core region by 8 Å to mimic an open clamp polymerase structure such as observed in cryo-EM studies of the eukaryotic OC [13] . The position of the calculated credible volumes for all our antenna dyes remained largely unchanged by this alteration, that is, changes were small compared with the size of the credible volumes and therefore all further discussion is based on the closed clamp state of the polymerase in accordance with single-molecule experiments on the bacterial OC [35] . Position of the transcription factors and DNA in the archaeal OC To determine the positions of TBP, TFB and the upstream TATA DNA in the OC, we assembled complexes where a fluorescent donor was attached to positions on or around the predicted binding region of TBP, namely ntDNA(−18), (−24), (−30) or (−37) to residue S71 of TBP and to residue G262 of TFB ( Fig. 1 , Methods). 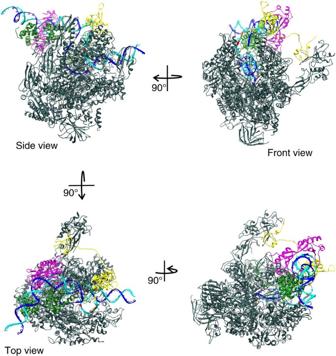Figure 5: Model of the complete archaeal OC. Side, front and top view and an alternate view obtained from the top view by a 90° rotation of the model of the open complex. DNA template and non-template strand are in blue and cyan, respectively. The transcription factors TBP, TFB and TFE are in purple, green and yellow, respectively. The ntDNA positions used for building the model are colour coded according to the NPS densities inFigs 3and4, namely ntDNA(+7), ntDNA(−1), ntDNA(−5), ntDNA(−7), ntDNA(−10), ntDNA(−12), ntDNA(−14), ntDNA(−18), ntDNA(−24), ntDNA(−30) and ntDNA(−37). The X-ray structure of the archaeal polymerase ofS. shibatae(PDB: 2WAQ; ref.37) is represented as a dark grey ribbon. See alsoSupplementary Fig. 8. Fluorescent acceptors were attached to one of the four reference sites on the RNAP, namely residues Rpo1′-G257, Rpo2″-Q373, Rpo7-V49 or Rpo7-S65, as before ( Supplementary Table 5 ). Residue K11 of Rpo5 was situated too far away to yield information for the localization process and was therefore left out from the analysis. The position of residues G44 in the winged-helix domain and G133 in the zinc ribbon domain of TFE had previously been determined by NPS [18] , and we included this smFRET data into the global NPS calculation to yield an accurate model of the complete archaeal OC ( Fig. 1 ). To maximize the resolution of the NPS, we used a valuable feature of the global analysis, which allows inclusion of FRET measurements between two unknown positions. We therefore included smFRET measurements from all the TATA DNA positions to both TBP and TFB and also smFRET measurements between TBP and TFB ( Fig. 1a dotted red lines and Supplementary Table 5 ). This procedure greatly increased the accuracy of all the determined dye positions. Corresponding histograms are shown ( Supplementary Figs 6g–l and 7 ). As a result of Bayesian parameter estimation, we obtained the three-dimensional probability density for the position of each antenna dye ( Fig. 4a–d ). Figure 4: Localization of the TATA DNA and transcription factors in the archaeal OC. ( a , b ) Side and front view of the archaeal RNA polymerase together with the NPS results for the fluorescent probes attached to ntDNA(−18) (dark cyan), ntDNA(−24) (dark blue), ntDNA(−30) (magenta), ntDNA(−37) (gold), TBP-S71 (purple), TFB-G262 (olive), TFE-G44 (yellow) and TFE-G133 (green). ( c ) Top view of archaeal RNA polymerase with only the NPS credible volumes TFE-G44 (yellow) and TFE-G133 (green) shown at a time to illustrate their proximity to the clamp coiled-coil region of subunit Rpo1′ (red) and to the stalk of the RNAP (black), respectively. ( d ) Alternative view obtained by a 90° rotation of the top view, showing the proximity of the NPS credible volume ntDNA(−18) (dark cyan) to the protrusion (brown) of subunit Rpo2″. The NPS credible volume of ntDNA(−24) (dark blue) is situated further away from the RNAP surface compared with the position of ntDNA(−18). Also, the proximity of the NPS credible volumes TBP-S71 (purple) and TFB-G262 (olive) to the wall domain (beige) of subunit Rpo2″ and to subunit Rpo12 (light blue) can be seen. The volume of TFB-G262 is made transparent for clarity. See also Supplementary Figs 6 and 7 . Full size image The credible volume for ntDNA(−18) ( Fig. 4d , dark cyan) is adjacent to the protrusion domain, and defines the path of the double-stranded ntDNA strand when compared with the position of the more downstream ntDNA(−14) and ntDNA(−12) ( Fig. 3c ), which are located further away towards the clamp domain. The first credible volume describing the position of the TATA box, ntDNA(−24) ( Fig. 4d , dark blue), is situated closer to the RNAP wall but further away from the RNAP surface compared with the position of ntDNA(−18). Together with the credible volume of the second TATA box position, ntDNA(−30) ( Fig. 4a,b , magenta), the bend in the DNA caused by TBP (centred at positions −26/−27) can be visualized. The credible volume of the last localized position on the ntDNA strand, ntDNA(−37) ( Fig. 4a,b , gold), is located adjacent to ntDNA(−30), indicating the upstream path of double-stranded DNA leading away from TBP. The position of residue S71 of TBP ( Fig. 4d , purple) is located between the credible volumes of ntDNA positions (−24) and (−30) and in proximity to the RNAP wall and subunit Rpo12 and is consistent with crystal structures of TBP in complex with DNA. The credible volume of TFB-G262 ( Fig. 4d , olive) is located further away from the protrusion domain than TBP and positioned closer to RNAP subunit Rpo12. For the localization of TFE, we used the previously published smFRET data in our global analysis. The global NPS localization for the two residues of TFE yields very similar positions than those determined previously [18] but the credible volumes are smaller due to the increased accuracy of the global NPS calculation ( Fig. 4c , yellow and green). This location of the TATA box in the archaeal OC is distinct from that previously determined in our group using NPS for a minimal eukaryotic OC [27] . In these studies a different promoter DNA sequence had been used (together with endogenous yeast Pol II and recombinant yeast transcription factors) and thus the question whether the particular conformation in an OC depends on the respective sequence arises [36] . We performed control measurements with a different DNA scaffold and concluded that the observed conformation is independent of the underlying promoter sequence, and as such our structural conclusions about the archaeal OC have general value ( Supplementary Fig. 8a and Supplementary Methods ), and that the differences compared with the earlier studies are due to the difference in the OC structure between yeast and archaea. Model of the complete archaeal open promoter complex To build a model of the complete archaeal RNAP OC, we started with the RNAP structure from Sulfolobus shibatae (PDB 2WAQ; refs 37 , 38 ) and used the calculated probability densities of the antenna dye attachment points on the ntDNA strand, TBP, TFB and TFE to position these elements and the tDNA onto this RNAP structure ( Fig. 5 ). To arrive at a unique structural model, we made some structural assumptions such as the size of the melted region, or the point of melting and re-annealing, all based on published data (see Methods for details). Figure 5: Model of the complete archaeal OC. Side, front and top view and an alternate view obtained from the top view by a 90° rotation of the model of the open complex. DNA template and non-template strand are in blue and cyan, respectively. The transcription factors TBP, TFB and TFE are in purple, green and yellow, respectively. The ntDNA positions used for building the model are colour coded according to the NPS densities in Figs 3 and 4 , namely ntDNA(+7), ntDNA(−1), ntDNA(−5), ntDNA(−7), ntDNA(−10), ntDNA(−12), ntDNA(−14), ntDNA(−18), ntDNA(−24), ntDNA(−30) and ntDNA(−37). The X-ray structure of the archaeal polymerase of S. shibatae (PDB: 2WAQ; ref. 37 ) is represented as a dark grey ribbon. See also Supplementary Fig. 8 . Full size image To estimate how well our new model fits the NPS probability densities, we calculated the accessible volume of the antenna dyes using the coordinates from our model of the archaeal OC. We found that in all but one case, the accessible volumes overlap with the corresponding NPS probability densities, showing that the built model is accurate (for more details see Methods). The smFRET and global NPS data presented here reveal the complete architecture of the open promoter complex in archaea including the paths of the ntDNA and tDNA strands, and the location of the three transcription initiation factors TBP, TFB and TFE. The resulting model provides a framework for understanding the molecular mechanisms of transcription initiation in the archaea, as well as allowing a comparison to the mechanism in the eukaryotic OC and providing insights into the evolution of the transcription machinery following the divergence of the archaeal and eukaryotic lineages. The formation of complete archaeal OCs was strictly dependent on TBP and TFB, and the overall architecture and in particular the path of the DNA was independent of its sequence. The DNA strands are melted and the tDNA strand has been loaded into the active centre cleft directly comparable to eukaryotic OCs [13] , [30] . In our model of the archaeal OC, the double-stranded downstream DNA enters the archaeal polymerase at a similar angle to that previously shown for structures in yeast, bacteria and archaea containing short duplex DNA [30] , [38] , [39] . In this position the downstream DNA can be stabilized by the proximal lysine-rich region of the jaw domain of Rpo1″ (residues 189–239), whereas the corresponding eukaryotic jaw domain would need a rotation inwards to superimpose with the archaeal counterpart, a movement hindered by the eukaryotic subunit Rpb9 and the N-terminal domain of the eukaryotic subunit Rpb5 that are not conserved in the archaeal RNAP [38] . The archaeal subunit Rpo5, which lacks the N-terminal domain of Rpb5, is required for the formation of stable OCs [40] and has been shown to photo-crosslink to the downstream DNA [41] , which is perfectly consistent with our model. Previously, we observed a dynamic switching of the downstream DNA into and out of the cleft in single-molecule studies of a minimal eukaryotic OC [27] . Cryo-EM data show that TFIIF appears to facilitate this transition in eukaryotes [13] . In contrast, in the archaeal OC, the smFRET data for ntDNA(+7) in the downstream double-stranded region showed no evidence of a dynamic movement of the DNA. Presumably, the transcription factor TFE, which is known to stabilize the DNA in the OC, renders the downstream DNA in a stable conformation. Note that the studies on the minimal eukaryotic OC were performed in absence of TFIIE. Thus it would be interesting to see whether the eukaryotic TFIIE has a similar function and would lead to a stabilization of the loaded state. Functional transcription assays using the Pol II system demonstrate that TFIIE stimulates OC formation and transcription on negatively supercoiled templates independent of TFIIH, which is in good agreement with our data and validates the use of archaeal transcription systems as bona fide model systems for eukaryotic Pol II (refs 42 , 43 ). In our model the downstream DNA strands are separated at register ntDNA(+2) in proximity to fork loop 2 (subunit Rpo2″, residues 436–445), and close to the highly conserved residue R446, which corresponds to Rpb2 residue R504 in Pol II. A point mutation of this arginine in the Pyrococcus RNAP (R445) to alanine leads to elongation deficiency in vitro [21] . Our model is also in agreement with the additional function of fork loop 2 of sterically blocking the duplex binding of the DNA and thus preventing re-association of the separated strands [44] . Therefore, at these positions, both tDNA and ntDNA strand conformations are very similar to those observed in the EC [26] . Further upstream, between registers ntDNA(−1) and (−7), the ntDNA strand runs adjacent to the fork loop 1 element (residues 404–410) and lobe domain of Rpo2″, the rudder of the Rpo1′ clamp (residues 278–297) and the linker region of TFB. Here the path of the ntDNA of the archaeal PIC diverges from that in the eukaryotic EC, as the TFB-linker region is situated at a position where it would clash with the ntDNA strand of the EC. NtDNA registers (−1) to (−3) pass close to the rudder, fork loop 1 and the TFB linker, whereas registers (−4) to (−7) are closer to the lobe. These protein interactions with the middle of the transcription bubble are highly likely to play a role in bubble melting and/or maintenance. Previous studies have shown the essential role of the Rpo1′ rudder in DNA strand separation, where mutants lacking this loop could not separate or maintain melted DNA [21] . In addition, yeast nuclear extracts containing temperature sensitive TFIIB were transcriptionally inactive in vitro and rescued only by adding recombinant wtTFIIB and not with TFIIB-containing mutations in the linker region [5] . Similarly, in vitro transcription assays with Pyrococcus furiosus RNAP and its initiation factors showed that point mutations or deletions in the TFB linker region allowed the formation of PICs but were inhibited for transcription [5] , and subsequent footprinting studies showed that these PICs were incapable of opening the promoter DNA. Thus, the B-linker region and Rpo1′ rudder are essential for promoter opening and OC stabilization. Our new model of the archaeal OC gives a mechanistic reason for these observations since the single-stranded ntDNA is positioned adjacent to all of these elements ( Fig. 6a,b ) and their interaction is likely to influence the stability and formation of the transcription bubble. 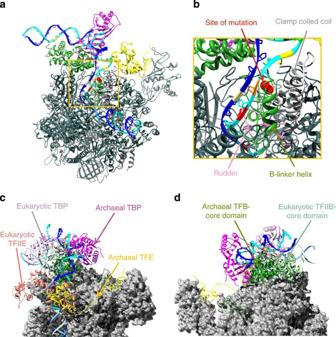Figure 6: Open complex model has implications for the melting of DNA in the CC to OC transition. (a) Side view (slightly rotated for a clearer view) of the archaeal polymerase ofS. shibatae(PDB: 2WAQ)37(dark grey) together with components of the open complex model, namely TFB, TBP as well as the template and non-template strand. (b) Detail of the yellow rectangular region inashowing the clamp coiled-coil domain of subunit Rpb1′ (light grey) and the point mutation introduced into the B-linker helix in a previous study (red)5. The rudder loop of Rpb1′ is shown in pink. (c,d) Detailed views of the archaeal model compared with the eukaryotic open complex model. The eukaryotic OC model5is displayed as superposition to the archaeal model and the archaeal RNAP. The eukaryotic transcription factors TBP and TFIIB are shown in light pink and light green, respectively. The DNA is shown in light blue and the polymerase is represented as a surface. For the archaeal OC model, the same colour coding is used as inFig. 5 Figure 6: Open complex model has implications for the melting of DNA in the CC to OC transition. ( a ) Side view (slightly rotated for a clearer view) of the archaeal polymerase of S. shibatae (PDB: 2WAQ) [37] (dark grey) together with components of the open complex model, namely TFB, TBP as well as the template and non-template strand. ( b ) Detail of the yellow rectangular region in a showing the clamp coiled-coil domain of subunit Rpb1′ (light grey) and the point mutation introduced into the B-linker helix in a previous study (red) [5] . The rudder loop of Rpb1′ is shown in pink. ( c , d ) Detailed views of the archaeal model compared with the eukaryotic open complex model. The eukaryotic OC model [5] is displayed as superposition to the archaeal model and the archaeal RNAP. The eukaryotic transcription factors TBP and TFIIB are shown in light pink and light green, respectively. The DNA is shown in light blue and the polymerase is represented as a surface. For the archaeal OC model, the same colour coding is used as in Fig. 5 Full size image As a consequence of the displacement of the ntDNA to the outside of the cleft relative to its path in the EC, its path comes close to the edge of the clamp core region and in particular to the clamp helix-coil-helix motif at register nt(−12) where the upstream end of the bubble lies. Previously, we have localized the binding position of the winged-helix domain of TFE [18] to the tip of the helix-coil-helix motif and the global NPS analysis presented in this paper also confirms this observation. Moreover, cryo-EM as well as crosslinking data show that eukaryotic TFIIE contacts the RNAP at a similar binding site [9] , [13] , [14] . Our model describes an interaction at this point between ntDNA at the upstream end of the bubble, TFE and the RNAP helix-coil-helix motif. These interactions are likely stabilizing the upstream end of the transcription bubble to prevent its collapse. The point of DNA re-annealing at register ntDNA(−12) lies above a tunnel formed by the N-terminal domain of the TFB core, the TFB-linker helix region, the rudder, the protrusion and TFE. A comparison to the position of the upstream DNA in the EC [26] shows that a rearrangement of the complete upstream double-stranded region, including a release of TFB core from the RNAP surface and movement of the upstream DNA to a position in between Rpo1′ helix α8 (residues 235–251) and Rpo2″ helix α11 (residues 349–373), is required during the initiation to elongation transition, presumably leading to a release of the transcription initiation factors and bubble collapse. Interestingly, the probability density for position ntDNA(−24), together with those for ntDNA(−30), ntDNA(−37), TBP-S71 and TFB-G262 define the pathway of the DNA strand around the TATA box in close proximity to the surface of the polymerase. Previous Far-Western blotting studies showed the strongest protein–protein interactions of TBP and TFB with subunits Rpo12, Rpo10 and Rpo2″ (ref. 45 ), which are all very close to the positions of the transcription factors in this OC model. Compared with the eukaryotic system, we find that the position of the TFB core domain in the archaeal OC has shifted and the position of TBP has changed substantially by ≈45 Å ( Fig. 6c,d and Supplementary Movie 1 ) [5] , [13] . While the N-terminal cyclin fold of the TFB core is only slightly tilted, the C-terminal cyclin fold of the TFB core is shifted and is localized closer to the DNA strand but still remains in proximity to the wall of the polymerase. Thereby, the helix-turn-helix motif consisting of helices TFB-H 4′ and TFB-H 5′ (residues K1265–K1292) is facing the ntDNA strand at registers ntDNA(−31) to ntDNA(−36), which form the purine-rich B-recognition element BRE. Mechanistically, transcription initiation in archaea is ancestral and streamlined compared with the eukaryotic Pol II system. Archaeal genomes do not encode homologues of TFIIA, TFIIF, TBP-associated factors and TFIIH. In particular the latter two could make important contributions to the OC formation since the TBP-associated factors make contact with the promoter DNA around the transcription start site, and TFIIH because of the ATP-dependent helicase/translocase activity is crucial for DNA melting on the majority of promoters tested in vitro and probably all transcription initiation in vivo [11] . However, using negatively supercoiled DNA and strong promoter templates, TBP and TFIIB suffice for initiation of eukaryotic Pol II (ref. 3 ), which demonstrates that the same ancestral mechanisms are able to facilitate OC formation in eukaryotes and archaea. Why are additional factors required by Pol II provided that the basic mechanisms are conserved? Our model of the complete archaeal OC provides a structural hypothesis for this apparent ease of DNA melting in archaea ( Fig. 7 ). Since the archaeal RNAP pulls the promoter-bound factors TBP and TFB much closer to its surface than Pol II ( Fig. 6c,d ) and the downstream promoter DNA is bound between the RNAP jaws, this topology likely induces a torsional strain in the DNA that lowers the local melting temperature of the promoter DNA. Interactions between the tDNA and residues on the inside of the DNA binding channel subsequently facilitate a swift loading of the tDNA strand into the RNAP active site. But why has this process evolved to become ATP energy dependent in the Pol II system while remaining spontaneous in archaea? Neither Pol I, nor Pol III, nor the bacterial sigma70 holo-RNAP requires energy for OC formation, which indicates that Pol II could be exceptional in this regard. Since the complexity of the Pol II transcriptome is higher than of any other RNAP system mentioned above, the energy dependence could reflect an additional layer of regulation of Pol II transcription. Support for this concept is provided by a recent report about the global regulation of OC formation in naïve lymphocytes [46] , which on activation undergo a transcriptome amplification that is regulated by TFIIH. 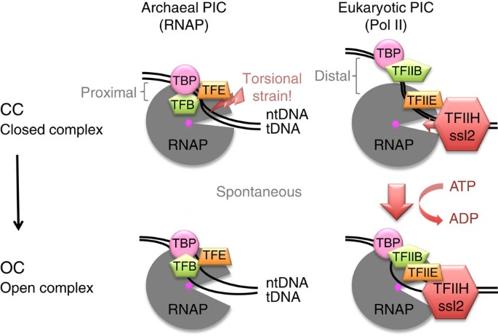Figure 7: Mechanisms of the closed to open complex transition in archaea and eukaryotes. During open complex formation the double-stranded promoter DNA is melted and the template DNA strand (tDNA) is loaded into the active site while the non-template strand (ntDNA) interacts with the RNAP clamp, and with TFE and TFIIE in archaea and eukaryotes, respectively (highlighted in orange). Concomitantly the entire complex—RNAP and initiation factors—undergoes large scale conformational changes. In archaea, OC formation occurs spontaneously and is possibly driven by the torsional strain in the promoter DNA induced by the interaction network between initiation factors, RNAP and the promoter DNA elements. While the upstream BRE and TATA promoter elements are anchored to the PIC by TFIIB (green) and TBP (magenta), the downstream DNA interacts with the RNAP jaws. In the Pol II system, OC formation is largely driven by the ATP hydrolysis-dependent activities of the TFIIH subunit ssl2 (red), which also induces a torsional strain by translocating the downstream promoter DNA in the upstream direction into the active site of RNAP. Figure 7: Mechanisms of the closed to open complex transition in archaea and eukaryotes. During open complex formation the double-stranded promoter DNA is melted and the template DNA strand (tDNA) is loaded into the active site while the non-template strand (ntDNA) interacts with the RNAP clamp, and with TFE and TFIIE in archaea and eukaryotes, respectively (highlighted in orange). Concomitantly the entire complex—RNAP and initiation factors—undergoes large scale conformational changes. In archaea, OC formation occurs spontaneously and is possibly driven by the torsional strain in the promoter DNA induced by the interaction network between initiation factors, RNAP and the promoter DNA elements. While the upstream BRE and TATA promoter elements are anchored to the PIC by TFIIB (green) and TBP (magenta), the downstream DNA interacts with the RNAP jaws. In the Pol II system, OC formation is largely driven by the ATP hydrolysis-dependent activities of the TFIIH subunit ssl2 (red), which also induces a torsional strain by translocating the downstream promoter DNA in the upstream direction into the active site of RNAP. Full size image In conclusion, the presented data provides a structural model for the organization of the archaeal OC. Given this model, a mechanism by which DNA melting could occur without transcription factor TFIIH becomes apparent. Recombinant protein preparation and labelling RNAP subunits from the hyperthermophilic archaeal model system M. jannaschii were expressed in recombinant form in Escherichia coli and purified [16] . For the smFRET experiments, five differently labelled RNAPs were prepared. Therefore, either single cysteine residues were introduced into the RNAP at position K11 of Rpo5 or positions V49 and S65 of Rpo7 and the subunits were purified and labelled with the dye Alexa647 (ref. 17 ). Or an unnatural amino acid ( p -Azido-L-phenylalanine) was introduced at position G257 of Rpo1′ and position Q373 of Rpo2″ and labelled with the dye DyLight650 by Staudinger ligation [47] . The fluorescently labelled subunits were directly introduced into RNAP reconstitution reactions following known protocols [16] . Unlabelled transcription factors TBP, TFB and TFE were expressed in recombinant form in E.coli [22] , [48] . TFE was labelled with either the dye Cy3B attached to position G44 or the dye DyLight550 attached to position G133 by Staudinger ligation [18] , [47] . Preparation of fluorescently labelled TBP derivative TBP was labelled with an Alexa647 or Alexa555 fluorophore via a cysteine–maleimide coupling strategy. To introduce a unique cysteine residue, the native cysteines at positions C48 and C67 that are buried inside the protein have been substituted by serine residues and a single cysteine residue has been introduced at position S71. The mutations have been introduced into the TBP gene using either the QuikChange II site-directed mutagenesis kit (Agilent) or the splice by overlap extension PCR strategy. Recombinant TBP-S71C was expressed from a pET21a(+) vector in BL21(DE3)/Rosetta cells and expression of TBP was induced in exponentially growing cultures with 1 mM isopropyl β-D-1-thiogalactopyranoside at an optical density of ~0.6 to 0.8 in rich medium for 4 h at 37 °C. Bacterial cells were harvested, resuspended and extracted in P300 buffer (200 mM Tris/acetate pH 7.9, 100 mM MgAc, 0.1 mM ZnSO 4 , 300 mM KAc, 10% glycerine). Cells were lysed using sonification. Recombinant and heat stable MjTBP could further be pre-purified using a heat denaturation step (65 °C for 20 min). The heat stable fraction contained MjTBP and the protein was precipitated with saturating amounts of ammonium sulfate. After pelleting the precipitated protein fraction, the pellet was resuspended in 5 ml P300 with 0.05% beta-ME and further purified by size exclusion chromatography (HiPrep-Sephacryl, S100 16/60, GE Healthcare). MjTBP containing fractions were combined, subsequently further purified and β-mercaptoethanol was removed by ion exchange chromatography (MonoQ 4.6/100 PE, GE Healthcare) using a gradient from 100 to 1,000 mM potassium acetate. The labelling reaction was carried out using a 10-fold molar excess of dye at 4 °C for 16 h. Labelled protein was separated from excessive free dye using a NAP-5-column and P100 buffer (200 mM Tris/acetate pH 7.9, 100 mM MgAc, 0.1 mM ZnSO 4 , 100 mM KAc, 10% glycerine) with 0.05% beta-ME. Preparation of fluorescently labelled TFB derivative For the production of fluorescently labelled TFB variants a nonsense-suppressor strategy was chosen, which allows the specific labelling of the protein via a unique unnatural amino acid (p-Azido-L-phenylalanine) [49] . An amber mutation (TAG) was introduced at position G262 into the TFB gene using the QuikChange II site-directed mutagenesis kit. The mutated protein was expressed from a pET21a(+) plasmid, which allowed purification of the full-length protein via a C-terminal His-tag. The recombinant protein was produced in BL21/DE3 cells that additionally carried the arabinose-inducible pEvolv-pAzF plasmid encoding multiple copies of an amber-suppressor tRNA (tRNA CUA ) and an engineered tyrosyl-tRNA synthetase [50] . Bacterial cultures were grown in rich medium containing 100 μg ml −1 ampicillin and 25 μg ml −1 chloramphenicol. p-Azido-L-phenylalanine (1 mM, Chem-Impex International Inc.) and 0.02% arabinose were added to the culture at an optical density of 0.3–0.4. TFB expression was induced with 1 mM isopropyl β- D -1-thiogalactopyranoside at an optical density of 0.5–0.6 and cells were harvested after 3 h. After harvesting the cells by centrifugation (5,000 g , 15 min), the cells were resuspended in N500 buffer (200 mM Tris/acetate pH 7.9, 100 mM MgAc, 0.1 mM ZnSO 4 , 500 mM NaCl, 10% glycerine) containing 0.5% Triton. Cells were lysed by sonification and the soluble protein fraction was extracted. The cell lysate was removed from cell debris and unsoluble fractions by a centrifugation step (15,000 g , 30 min) and the supernatant was further purified by affinity chromatography (HisTrap FF 1 ml, GE Healthcare). Following labelling with 10-fold molar excess of either DyLight550 or DyLight650 via Staudinger ligation [47] overnight at 4 °C, the excess of free dye was removed by affinity chromatography (HisTrap FF 1 ml). KMnO 4 footprinting The DNA template encoding the SSV T6 promoter was prepared by annealing 5′, 32 P-labelled ntDNA strand (5′-GATTGATAGAGTAAAGTTTAAATACTTATATAGAT AGAGTATAGATAGAGGGTTCAAAAAATGGTT-3′) and unlabelled tDNA strand (5′-AACCATTTTTTGAACCCTCCGCTTATACTCTATCTATATAAGTATTTAAACTTTACTCTATCTATC-3′). For the footprinting reactions, the components were combined in 23 μl reactions containing 1 × HNME buffer (40 mM HEPES (pH 7.3), 250 mM NaCl, 2.5 mM MgCl 2 , 0.02 mM EDTA, 1% glycerol and 2 mM DTT), 8.3 nM tDNA, 0.6 μM RNAP, 8.7 μM TBP, 0.5 μM TFB and 740 nM TFE. The reaction was incubated at 65 °C for 15 min followed by a 2-min incubation with 2 μl KMnO 4 (at 4, 8 or 16 mM) and stopped with 1.5 μl 14 M β-ME. Protein was digested by addition of 0.25% SDS and 1 mg ml −1 proteinase K and incubation at 65 °C for 1 h. DNA was ethanol precipitated prior to treatment with 5% piperidine at 90 °C for 30 min, followed by one round of chloroform extraction and subsequent ethanol precipitation. To prepare the A+G ladder, the DNA was treated with formic acid for 5 min prior to DNA precipitation and piperidine treatment as described above. DNA was separated on 10% urea PAGE, exposed to a phosphor storage screen and visualized on a Typhoon FLA 9500 bioimager. Archaeal OC preparation for single-molecule FRET experiments The OCs were assembled freshly before each smFRET experiment by adding 1 μl each of nucleic acid scaffold (2 μM), TBP (10 μM), TFB (10 μM), RNAP ΔRpo4/7 (2 μM) and Rpo4/7 (10 μM) to 10 μl HNME buffer. The mixture was incubated at 60 °C for 10 min. Heparin (final concentration 0.5 mg ml −1 ) was added to reduce non-specific binding of the RNAP to nucleic acids. Unbound transcription factors and nucleic acids were removed using Amicon Ultra centrifugal filters (Millipore) by washing two times with 450 μl HNME buffer. All smFRET experiments were done in presence of TFE (12 μM), which was added to the purified complexes and incubated for 10 min at 60 °C. The complexes were then diluted 1,000-fold in HNME buffer and loaded into the sample chamber of the TIRF microscope. For surface immobilization of the complexes, the ntDNA strand had biotin attached at the 5′-end via a C6-amino linker. The DNA single-strands were purchased from IBA (Göttingen, Germany) and annealed as described before [25] . The viral SSV T6 promoter DNA [51] was used for all the smFRET experiments as it is known to form very stable PICs in promoter-directed transcription in vitro [16] . Our promoter DNA constructs consists of a 66-nucleotide long double-stranded DNA with tDNA and ntDNA strands containing a 4 nucleotide heteroduplex region around the transcription start site (−3 to +1) that stabilized the PIC by forming the OC ( Fig. 1 ). For the determination of the course of the ntDNA within the OC, the ntDNA strand was purchased with either Cy3B at position (+7), (−1), (−5), (−7), (−10), (−12), (−14), (−18), (−30) and (−37) or 6-TAMRA at position (−24) ( Fig. 1b ). For the question of the conformation of the tDNA in the OC, the tDNA strand was purchased with 6-TAMRA at position (+3) and Cy3B at position (−9). Experimental set up for smFRET and data analysis All smFRET experiments were performed on a custom-built prism-based total internal reflection fluorescence microscope [18] . Briefly, a frequency-doubled Nd:YAG laser (532 nm, Spectra-Physics) was used for the excitation of donor molecules and a diode laser (643 nm, Toptica) for the direct excitation of the acceptor molecules. Fluorescence intensity was collected through a water immersion objective (Plan Apo × 60, numerical aperture 1.2, Nikon) and directed to an EMCCD camera (iXon, Andor). OCs were immobilized onto the surface of a microfluidic chamber surface via PEGBiotin–Neutravidin–Biotin [25] . The acquired data was analyzed using custom-written MATLAB software. We used a fully automated routine to find FRET pairs, calculating and subtracting the local background and computing the fluorescence trajectories [25] . The correction factors were determined individually for every FRET pair. The resulting histograms were computed for every time point (frame-wise histogram). Data from at least three individual smFRET measurements were used for each pair of labelling sites. The FRET efficiencies from all molecules of all measurements were plotted in histograms. The peaks were fitted with one (or two) Gaussian function(s) to extract the mean FRET efficiencies ( Supplementary Tables S1, S4 and S5 ). A s.d. of 2% for the FRET efficiencies was included into the calculation. These results were then used for further analysis with NPS [24] or global NPS [28] , as indicated. Determination of the probability densities using NPS The X-ray structure of the archaeal RNAP of S. shibatae (pdb file: 2WAQ; ref. 37 ) was used as a reference frame for the position calculation. Moreover, the volume occupied in the crystal structure was used as a restriction for the possible positions of the dye molecules. We assumed zero probability density within an already occupied volume, which was the volume of the protein shrunk by 5 Å to account for uncertainties in the X-ray structure and equal probability density elsewhere to calculate the ADM prior. The global NPS method [28] , software freely available at http://www.uni-ulm.de/nawi/nawi-biophys/software.html ) was then applied using the available X-ray structures, the measured FRET efficiencies and Bayesian parameter estimation. As a result, we obtained the three-dimensional probability density function for the positions (+7), (−1), (−5), (−7), (−10), (−12), (−14), (−18), (−24), (−30) and (−37) on the ntDNA strand, as well as the positions of residue S71 of TBP and residue G262 of TFB. From this we calculated the smallest volumes that enclose a certain probability, so-called credible volumes. The surface of the credible volumes was displayed by using the interactive visualization programme UCSF Chimera, which was also used for displaying all structural data [52] . All credible volumes shown in the paper are calculated at 68% probability. For more details see Methods. Determination of isotropic Förster radii and anisotropies For each donor–acceptor pair, the isotropic Förster radius R 0 iso was determined using standard procedures [53] . First, the quantum yield (QY) of the donor sample was determined using Rhodamine 101 dissolved in ethanol as a standard (QY=91.5%) [54] ( Supplementary Table 2 ). The ntDNA positions (+7), (−1), (−5), (−7), (−10), (−12), (−14), (−18), (−24), (−30) and (−37) were labelled either with the donor dye Cy3B or 6-TAMRA, residue S71 of TBP was labelled with the dye Alexa555 and residue G262 of TFB was labelled with the dye DyLight550. Second, overlap integrals were calculated from recorded donor emission spectra (528–700 nm with an excitation wavelength of 523 nm) and acceptor absorption spectra (400–700 nm). Together with the refractive index ( n =1.35) and the orientation factor ( κ 2 =2/3), the isotropic Förster radii R 0 iso were determined for all the different donors and Alexa647 as acceptor ( Supplementary Table 2 ). To account for uncertainties in the Förster distance due to orientation effects, we then measured the steady state fluorescence anisotropies of the donor and acceptor dyes for all attachment sites using a steady state fluorescence spectrometer (Edinburgh Instruments F900) ( Supplementary Table 2 ). Both, isotropic Förster distances as well as fluorescence anisotropies were used as prior information in the global NPS analysis [28] . Uncertainty in the position of satellite dye molecules Satellite dye molecules (SDMs) were attached to known positions within the archaeal polymerase using flexible linkers. While the attachment point is known from the X-ray structure of the archaeal polymerase of S. shibatae (pdb file: 2WAQ; ref. 37 ), the precise location of the dye molecule is not. For the NPS analysis, we therefore calculated the volume that is sterically accessible to the dye molecules, given the point of attachment, size of the dye molecule and the linker length [24] . To this end, the SDMs were approximated by a sphere of diameter d dye and linked to the protein complexes by flexible linkers of dimensions L linker and d linker ( Supplementary Table 3 ). We assume that each SDM position within this accessible volume is equally probable ( Supplementary Fig. 4 ). Calculation of model-based prior volumes For the dyes attached to the double-stranded DNA region, the coordinates of the C7 atom of the base were used as attachment point and the linker length corresponded to 12 C-atoms. In case of the single-stranded ntDNA region, the base orientations were left out of the model, since in a single strand of nucleic acids base stacking energies are small and as a result any base is relatively free to rotate about the backbone. Therefore, a 17 C-atom linker and an attachment point on the backbone C1′ atom of the DNA was used for single-stranded regions. The sequence alignment of the proteins TBP and TFB from M. jannaschii that were used in all our experiments with the corresponding proteins from P. woesei contained in the crystal structure of the TBP/TFB/DNA sub-complex used for the modelling (pdb file: 1D3U; ref. 51 ) resulted in the definition of the analogous residues S72 for TBP and E1223 for TFB in the model. Exemplary Figures of the comparisons can be found in Supplementary Fig. 8b–e . Modelling A number of structural assumptions were made to arrive at a unique model: (1) The extent of the single-stranded transcription bubble is between positions (−11) and (+1), corresponding to the permanganate footprinting results and published literature [5] , [32] , [33] . (2) The tDNA strand position (+1) would be positioned at the active site for base pairing with the first NTP of the RNA transcript. (3) The DNA conforms to a B-form duplex outside of the melted region, and the downstream duplex occupies a similar position to that of the eukaryotic/bacterial EC [44] , [55] , the OC-mimic of Pol II (ref. 30 ) and the archaeal RNAP-DNA binary complex [38] . (4) The structure of archaeal TBP/TATA/TFB from P. woesei (PDB 1D3U; ref. 51 ) containing the C-terminal cyclin core of TFB and a bent TATA box DNA fragment was used as the template for TBP–TATA–TFB in this OC model and would not change in conformation when bound to RNAP. (5) The path of the TFB N-terminal regions within the RNAP cleft would follow the same approximate path as observed in the structure of eukaryotic Pol II in complex with TFIIB (PDB 4BBR; ref. 7 ). (6) The position of the N- and C-terminal domains of TFE would also be consistent with the cryo-EM density observed for the eukaryotic Pol II PIC containing TFIIE (ref. 13 ). Probability densities were visualized in Coot [56] and USCF Chimera [52] . Template models assembled into the complete OC model were based on PDB entries 2WAQ, 1D3U, 4BBR, 1Q1H and 1VD4. Models were manipulated to fit the probability densities using the same programmes as for visualization, and geometry was regularized using phenix.refine [57] . Model coordinates are given in a Supplementary File . To estimate how well the model fits the NPS densities, we calculated the accessible volume priors of the dyes attached to the respective positions in the model (Methods) and compared them with our resulting probability densities. It should be noted that a perfect overlap is not expected given the nature of the model-based prior and the NPS posterior. The prior volume encompassing the complete volume of the dye molecule could be sitting, given its size and the length of the linker and the position of the anchor point defined by the model of the OC. Therefore, its size is simply a measure of the uncertainty before the measurement. The posterior volume, in contrast, represents the probability for the dye position and its size is a measure of the uncertainty after the measurement. As long as there is overlap between prior and posterior, the model is in accordance with the data. The model and the derived accessible volumes fit the obtained credible volumes from the NPS calculation drawn at 68% credibility in all but one case ( Supplementary Fig. 8b,c ), the exception being the ntDNA(−14) position, where the calculated accessible volume is not overlapping with the computed NPS volume drawn at 68% credibility. The clamp coiled-coil region of the RNAP is situated exactly in between the accessible volume and the NPS credible volume of ntDNA(−14). If the NPS credible volume of ntDNA(−14) is displayed at 90% confidence level, the prior and posterior overlap ( Supplementary Fig. 8d,e ). One should note that TFE also binds to the clamp coiled-coil region as determined by previous cryo-EM, crosslinking and NPS studies [9] , [13] , [18] . However, we did not assign a particular volume for TFE in the NPS analysis. Thus, it is quite likely that large parts of the NPS determined credible volumes for the dye attached to ntDNA(−14) are in fact excluded by TFE, preventing overlap between the model and the NPS result for ntDNA(−14). How to cite this article : Nagy, J. et al. Complete architecture of the archaeal RNA polymerase open complex from single-molecule FRET and NPS. Nat. Commun. 6:6171 doi: 10.1038/ncomms7161 (2015).